Quality control of spliced mRNAs requires the shuttling SR proteins Gbp2 and Hrb1 Eukaryotic cells have to prevent the export of unspliced pre-mRNAs until intron removal is completed to avoid the expression of aberrant and potentially harmful proteins. Only mature mRNAs associate with the export receptor Mex67/TAP and enter the cytoplasm. Here we show that the two shuttling serine/arginine (SR)-proteins Gbp2 and Hrb1 are key surveillance factors for the selective export of spliced mRNAs in yeast. Their absence leads to the significant leakage of unspliced pre-mRNAs into the cytoplasm. They bind to pre-mRNAs and the spliceosome during splicing, where they are necessary for the surveillance of splicing and the stable binding of the TRAMP complex to spliceosome-bound transcripts. Faulty transcripts are marked for their degradation at the nuclear exosome. On correct mRNAs the SR proteins recruit Mex67 upon completion of splicing to allow a quality controlled nuclear export. Altogether, these data identify a role for shuttling SR proteins in mRNA surveillance and nuclear mRNA quality control. mRNA splicing is a characteristic feature of eukaryotic cells and enabled the development of multicellular organisms. However, the emergence of intron sequences required the simultaneous genesis of a nuclear envelope and the establishment of quality control systems that ensure the selective export of fully processed mRNAs. Results of failure on a single cellular level could be adecreased viability or in multicellular organisms diseases like cancer or neurodegenerative diseases [1] . At all levels of nuclear mRNA maturation, during transcription, splicing or 3′-end processing defective mRNAs can be produced, but are then caught and eliminated by the nuclear surveillance machinery [2] , [3] , [4] , [5] . Although only little is known about the underlying mechanisms, degradation of faulty mRNAs requires the nuclear exosome that contains a specific nuclear ribonuclease Rrp6 in addition to a nine-subunit exosome core associated with the 3′–5′ exoribonuclease Dis3/Rrp44 (refs 6 , 7 , 8 ). Moreover, the exosome requires co-factors such as the TRAMP complex ( Tr f4/ A ir2/ M tr4 P olyadenylation) that marks faulty mRNAs for degradation [4] , [9] . It consists of a poly(A) polymerase (Trf4 or Trf5), a Zn knuckle-containing RNA binding protein (Air1 or Air2) and the RNA helicase Mtr4 (refs 5 , 8 ). Consistently, inactivation of the TRAMP/exosome system leads to the accumulation of aberrantly or slowly processed pre-mRNAs [10] . In addition to its role in RNA quality control the TRAMP complex was suggested to degrade intron sequences and it was recently shown that it influences splicing [11] , [12] . How mRNAs are recognized as incorrect is still unclear, however, the nuclear pore complex (NPC) proteins Mlp1, Mlp2, Nup60 and Pml39 as well as the nuclear envelope protein Esc1 and the pre-mRNA retention and splicing complex protein Pml1 may play a role as their absence or mutations in their genes lead to the leakage of unspliced mRNAs into the cytoplasm [2] , [5] . Another exosome adapter was identified in mammalian cells and termed the nuclear exosome targeting (NEXT) complex, which is required for the degradation of non-coding transcripts [13] . It contains MTR4, an RNA-binding motif containing protein, RBM7 and the zinc finger CCHC domain-containing protein 8 (ZCCHHC8). Both, RBM7 and ZCCHHC8 co-purify with members of the serine/arginine (SR) protein family [13] , [14] . These findings link the SR proteins, which are known for their function in splicing, with the exosome and its co-factors, important for RNA degradation and it was suggested that the SR proteins might assist the NEXT complex in higher eukaryotes [3] . However, a direct involvement of the SR proteins in mRNA surveillance and a mechanism of how they might regulate quality control has not been shown yet. Splicing in yeast, analogous to higher eukaryotes, can be separated into early and late phases in which a number of proteins and ribonucleoparticles (snRNPs) associate and dissociate [15] . Notably, constitutive and alternative splicing in higher eukaryotes depend on SR proteins most of which are exclusively localized to the nucleus. Only few of them accompany the mature mRNAs to the cytoplasm [16] . In yeast, three SR-like mRNA-binding proteins exist, termed Npl3, Gbp2 and Hrb1, which shuttle from the nucleus to the cytoplasm when bound to the mature mRNA molecules [17] , [18] , [19] . All three yeast SR proteins are recruited to the mRNAs co-transcriptionally, Npl3 early by RNA polymerase II and Gbp2 and Hrb1 via the THO complex, a tetrameric complex consisting of Hpr1, Tho2, Mft1 and Thp2, that associates with the elongating RNApolymerase and has been implicated in transcription elongation, mRNA export and genome stability [5] , [17] , [20] , [21] . Upon mRNA maturation, Npl3 and in higher eukaryotes the three shuttling SR proteins (SRSF1, SRSF3 and SRSF7) have been suggested to function as adapters between the mRNA and the export receptor Mex67 (TAP/NXF1 in higher eukaryotes) to promote mRNA export to the cytoplasm [16] . Here we identify the SR proteins Gbp2 and Hrb1 as two novel quality control factors for spliced mRNAs. Our data suggest that they retain pre-mRNAs either until splicing is completed or until faulty mRNAs are degraded. For elimination of faulty mRNAs Gbp2 and Hrb1 associate with the TRAMP complex that guides those pre-mRNAs to the exosome. On correctly spliced mRNAs Gbp2 and Hrb1 instead recruit Mex67 to allow a quality controlled nuclear export. Splicing factor mutants prevent Gbp2 and Hrb1 nuclear export All three mammalian shuttling SR proteins and yeast Npl3 have been shown to interact with the export receptor TAP/Mex67 (ref. 16 ). To investigate whether the other two shuttling SR proteins in yeast, Gbp2 and Hrb1, also interact with Mex67 we performed in vivo co-immunoprecipitation (IP) experiments and found physical, RNase-insensitive interactions of all three yeast SR proteins and Mex67 ( Fig. 1a and Supplementary Fig. 1a,b ). Together with our previous finding showing that the export of Gbp2, Hrb1 and Npl3 is blocked in a mex67 mutant (ref. 17 and Fig. 1b ), these data indicate that all SR proteins utilize Mex67 as an export receptor. However, an interesting question is why does a cell need several different Mex67 adapter proteins? It seems likely that they have additional individual functions. 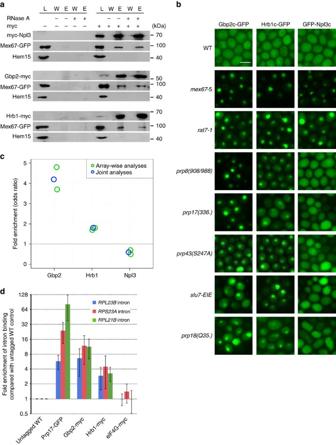Figure 1: Gbp2 and Hrb1 bind to Mex67 and require the functional spliceosome for their export. (a) The export receptor Mex67 physically interacts with all three SR proteins. Co-immunoprecipitation (IP) experiments were performed in cells expressing myc-tagged Npl3, Gbp2 or Hrb1. Log phase cells were lysed and split in two equal parts one of which was treated with RNase A (+/−). Hem15 served as a negative control. (L=lysate, W=final wash, E=eluate). (b) The export of Gbp2 and Hrb1 is dependent on splicing. At steady-state cytoplasmic versions of the GFP-tagged SR proteins (Gbp2c-GFP, Hrb1c-GFP, GFP-Npl3c) were produced in the indicated strains. Log phase cells were shifted to 37 °C for 30 min prior to fluorescence microscopy. Scale bar, 5 μm. (c) Microarray analyses from mRNAs that were co-immunoprecipitated with the myc-tagged SR-proteins reveal an enriched binding of Gbp2 and Hrb1 to intron-containing transcript. Shown is the enrichment of the intron-containing genes in the eluates relative to their expression level in the lysates. The fold enrichment is expressed in terms of the odds ratio, that is, the odd of being an intron gene among the bound genes in the eluate versus the unbound genes. Green circles show the values for individual arrays and blue circles those derived from joint analyses using linear models. (d) Gbp2 and Hrb1 bind to intron-containing transcripts. RNA co-IP experiments were performed with Prp17–GFP (positive control), myc-tagged Gbp2 and Hrb1 and the cytoplasmic translation factor eIF4G-myc (negative control). The co-precipitated RNA was used in qRT–PCR experiments to investigate the presence of three different intron sequences. Error bars represent the s.d. Figure 1: Gbp2 and Hrb1 bind to Mex67 and require the functional spliceosome for their export. ( a ) The export receptor Mex67 physically interacts with all three SR proteins. Co-immunoprecipitation (IP) experiments were performed in cells expressing myc-tagged Npl3, Gbp2 or Hrb1. Log phase cells were lysed and split in two equal parts one of which was treated with RNase A (+/−). Hem15 served as a negative control. (L=lysate, W=final wash, E=eluate). ( b ) The export of Gbp2 and Hrb1 is dependent on splicing. At steady-state cytoplasmic versions of the GFP-tagged SR proteins (Gbp2 c -GFP, Hrb1 c -GFP, GFP-Npl3 c ) were produced in the indicated strains. Log phase cells were shifted to 37 °C for 30 min prior to fluorescence microscopy. Scale bar, 5 μm. ( c ) Microarray analyses from mRNAs that were co-immunoprecipitated with the myc-tagged SR-proteins reveal an enriched binding of Gbp2 and Hrb1 to intron-containing transcript. Shown is the enrichment of the intron-containing genes in the eluates relative to their expression level in the lysates. The fold enrichment is expressed in terms of the odds ratio, that is, the odd of being an intron gene among the bound genes in the eluate versus the unbound genes. Green circles show the values for individual arrays and blue circles those derived from joint analyses using linear models. ( d ) Gbp2 and Hrb1 bind to intron-containing transcripts. RNA co-IP experiments were performed with Prp17–GFP (positive control), myc-tagged Gbp2 and Hrb1 and the cytoplasmic translation factor eIF4G-myc (negative control). The co-precipitated RNA was used in qRT–PCR experiments to investigate the presence of three different intron sequences. Error bars represent the s.d. Full size image In an attempt to identify specific functions for the SR proteins, we screened for factors that inhibit the nuclear export of a Gbp2 variant (Gbp2 c -GFP), which is impaired in the speed of nuclear import and thus is equally distributed in both compartments at steady state [17] . We identified several late splicing factor mutants that all block the export of Gbp2 ( Fig. 1b ). A similar export block is also detectable in strains producing an Hrb1–GFP fusion protein under the control of the strong ADH1 promoter that is mostly cytoplasmic at steady state (Hrb1 c –GFP). The nuclear localization in splicing factor mutants is not due to differences in the expression level of the protein ( Supplementary Fig. 1c ). In sharp contrast, we find that the export of a similarly cytoplasmic variant of Npl3, mutated in the Mtr10-binding domain (GFP-Npl3 c ), is not affected in these splicing factor mutants, whereas its export is impaired in mex67-5 or the nucleoporin mutant rat7-1 cells ( Fig. 1b ). Interestingly, for Npl3 an involvement in spliceosome assembly and the interaction with early splicing factors has been reported [22] , which suggested that the recruitment of the spliceosome might depend on Npl3. In contrast to that, the pre-mRNA association of Gbp2 and Hrb1 seems to be dependent on splicing ( Fig. 1b ). It has recently been published that the TREX complex interacts with the Prp19 complex, involved in splicing and transcription elongation and that it might recruit the TREX complex to mRNAs [23] . In fact, for spliced transcripts it has been shown earlier that pre-mRNA splicing seems to enhance the THO complex recruitment and THO complex components have been shown to stably bind to the mRNP after the second step of splicing [24] . As Gbp2 and Hrb1 are associated with this complex, it is possible that their recruitment is disturbed because the TREX complex recruitment is inhibited in splicing factor mutants. Although an association of Gbp2 and Hrb1 with spliced and unspliced transcripts determined by PCR amplification of co-immunoprecipitated mRNAs has been reported earlier [20] , their exclusive nuclear localization in splicing factor mutants suggests that they differ from Npl3 that bind to bulk mRNA and thus do not show export defects in splicing factor mutants [18] , [25] . Therefore, we investigated whether the two SR proteins preferentially bind spliced transcripts in genome wide analyses. We immunoprecipitated the myc-tagged SR proteins, purified the associated poly(A) + RNAs and applied them onto microarrays. Significantly, we detect an ~4.2-fold and 1.8-fold increased association of transcripts derived from intron-containing genes for Gbp2 and Hrb1, respectively, as compared with the intronless genes on the microarray, while no enrichment (0.6-fold) was found for Npl3 ( Fig. 1c ). Moreover, the microarray data reveal an increased binding of Gbp2 (30%) and Hrb1 (19%) to rRNA processing, ribosome biogenesis factors and highly expressed ribosomal protein genes, which is not the case for Npl3 ( Supplementary Fig. 1d ). That Npl3 rather binds to bulk mRNAs was also published earlier [26] . Furthermore, in support of our data, a preferential association of Gbp2 with unspliced transcripts was recently also identified by a transcriptome-wide technique termed CRAC (crosslinking and analysis of cDNA) [27] . These microarray data were verified by the direct analysis of three highly expressed intron-containing and intronless transcripts of the first hits of each microarray in qRT–PCR experiments. Interestingly, we found that only transcripts from intron-containing genes were enriched for Gbp2 and Hrb1, while Npl3 showed a generally high binding to bulk transcripts ( Supplementary Fig. 1e ), supporting a preferential association of Gbp2 and Hrb1 with intron-containing mRNAs. To investigate whether Gbp2 and Hrb1 are bound to intron-containing transcripts at early stages when the intron is still present, we performed RNA co-immunoprecipitation (RNA-IP or RIP) experiments with Prp17-GFP, Gbp2-myc, Hrb1-myc and the translation factor eIF4G-myc and found that similar to Prp17 and in contrast to eIF4G, Gbp2 and Hrb1 bind the intron sequences of RPL23B , RPL21B and RPS23A ( Fig. 1e and Supplementary Fig. 1f ), indicating that Gbp2 and Hrb1 are recruited to intron-containing transcripts at early stages when the intron is still present. In fact, Gbp2 and Hrb1 have been purified earlier with the activated B complex (B act ) of the yeast spliceosome [28] , indicating that they are associated with actively spliced mRNAs. Together, these results show that Gbp2 and Hrb1 have a preference to bind to transcripts derived from intron-containing genes and both SR proteins might selectively accompany those matured mRNAs derived from intron-containing genes to the cytoplasm. Gbp2 and Hrb1 interact with late splicing factors Owing to the fact that the export of Gbp2 and Hrb1 in late splicing factor mutants is prevented, we investigated potential genetic and physical interactions of the SR proteins with late splicing factors and compared these to Npl3. Indeed, we find that the combination of gbp2 Δ or hrb1 Δ single deletions with prp8 , prp17 and prp43 mutants show an impaired growth phenotype, their combination with the gbp2 Δ hrb1 Δ double knock out is in all cases even synthetically lethal ( Fig. 2a ). In contrast, we find no synthetic growth defects of npl3 Δ with these late splicing factors, although npl3 Δ is already impaired in growth. Interestingly, Kress et al. [22] detected no influence of gbp2 Δ in early splicing events, while npl3 Δ showed synthetic lethal interactions with early splicing factors. This is consistent with the idea of an early function of Npl3 by recruiting early splicing factors to the intron-containing pre-mRNAs and a later function for Gbp2 and Hrb1 during splicing. 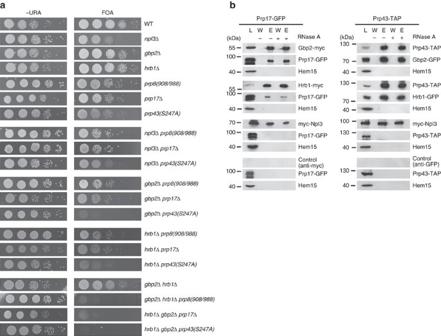Figure 2: Genetic and physical interactions of Gbp2 and Hrb1, but not Npl3 with late splicing factors. (a) Combinations ofgbp2Δhrb1Δ with splicing factor mutants are synthetically lethal. All mutants, containing covering plasmids encoding splicing factor genes orNPL3were spotted in serial dilution onto-uracil (URA) plates and onto 5′fluoorotic acid (FOA) plates that select for the loss of the covering plasmid. (b) Gbp2 and Hrb1 physically interact with splicing factors. Co-IP experiments were performed with myc-tagged Gbp2, Hrb1, Npl3 and Prp17-GFP (left) or Prp43-TAP (right). Log phase cells were lysed and split in two equal parts one of which was treated with RNase A (±). Hem15 served as a negative control. L, lysate; W, final wash; E, eluate. Figure 2: Genetic and physical interactions of Gbp2 and Hrb1, but not Npl3 with late splicing factors. ( a ) Combinations of gbp2 Δ hrb1 Δ with splicing factor mutants are synthetically lethal. All mutants, containing covering plasmids encoding splicing factor genes or NPL3 were spotted in serial dilution onto-uracil (URA) plates and onto 5′fluoorotic acid (FOA) plates that select for the loss of the covering plasmid. ( b ) Gbp2 and Hrb1 physically interact with splicing factors. Co-IP experiments were performed with myc-tagged Gbp2, Hrb1, Npl3 and Prp17-GFP (left) or Prp43-TAP (right). Log phase cells were lysed and split in two equal parts one of which was treated with RNase A (±). Hem15 served as a negative control. L, lysate; W, final wash; E, eluate. Full size image To further analyse whether also physical interactions between Gbp2 or Hrb1 and late splicing factors are detectable, we conducted co-IP experiments with myc- or GFP-tagged Gbp2 and Hrb1 and components of the spliceosome. We found physical, RNA independent interactions between Gbp2 or Hrb1 and Prp17 or Prp43 ( Fig. 2b ). In contrast, Npl3 showed no physical interactions with these splicing factors ( Fig. 2b ) [22] . Together, these data support the idea that both proteins might be recruited at later stages of splicing. To investigate whether these proteins have a function in the splicing process itself, we performed northern blot analyses with an intron-containing reporter gene and found in comparison to splicing factor mutants only very slight accumulations of unspliced transcripts for all three SR protein deletions ( Supplementary Fig. 2 ), which might be due to secondary effects, for example, a disturbed cross-talk between splicing and export or defects in the export-competence approval. These rather slight effects on splicing suggest that Gbp2, Hrb1 and Npl3 might not act as bona fide splicing factors. Stable binding of Gbp2 and Hrb1 to mRNAs and Mex67 depends on splicing Together, all data indicate a model in which Npl3 associates with bulk mRNAs, recruited by RNA polymerase II [21] , [26] . In case of the intron-containing transcripts it participates in the recruitment of the early spliceosome [22] . In contrast to that, Gbp2 and Hrb1 are loaded onto pre-mRNAs via the THO complex [17] , [20] ; however, a stable mRNA association might require splicing. Thus, we performed RNA co-IP experiments with the myc-tagged SR proteins and found that significantly less poly(A) + RNA was co-precipitated in three different splicing factor mutants in relation to the existing poly(A) + RNA in wildtype, while the amount of Npl3 associated mRNAs was nearly unaffected ( Fig. 3a and Supplementary Fig. 3 ). Similar to Npl3, the THO complex is recruited to bulk mRNA [25] . To see whether this would also be reflected in the RNA co-IP experiment we precipitated Tho2 and Thp2 and analysed their binding to poly(A) + RNA. Indeed, binding of these proteins to poly(A) + RNA only slightly depends on splicing, to a similar extend as seen for Npl3 and in contrast to Gbp2 and Hrb1 ( Fig. 3a ). These findings indicate that splicing is a prerequisite for the stable transcripts binding of Gbp2 and Hrb1. 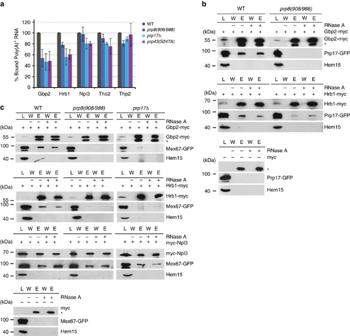Figure 3: Stable association of Gbp2 and Hrb1 with spliced mRNAs and Mex67 requires splicing and the interaction with splicing factors. (a) Significantly reduced association of Gbp2 and Hrb1 to poly(A)+RNAs in splicing factor mutants. RNA co-immunoprecipitation experiments were performed with myc-tagged Gbp2, Hrb1 and Npl3 and GFP-tagged Tho2 and Thp2 in the indicated strains shifted to 37 °C for 30 min in three independent experiments. The co-precipitated poly(A)+RNA was detected by northern dot-blot hybridizations with a digoxigenin-labelled oligo d(T)50probe, set into relation with the total mRNA present in each strain and quantified relative to wild type. Error bars reflect s.d. (b) Functional Prp8 is required for proper association of Gbp2 and Hrb1 with Prp17. Co-IPs with myc-tagged Gbp2 or Hrb1 and Prp17-GFP were performed in wild type andprp8(908/988)cells; *, antibody chain. (c) Splicing is required for recruitment of Mex67 to Gbp2 and Hrb1. Western blots show the interaction between myc-tagged Gbp2, Hrb1 or Npl3 and Mex67-GFP in the indicated strains. All strains were shifted to 37 °C for 30 min. (*, antibody chain; L=lysate, W=final wash, E=eluate). Figure 3: Stable association of Gbp2 and Hrb1 with spliced mRNAs and Mex67 requires splicing and the interaction with splicing factors. ( a ) Significantly reduced association of Gbp2 and Hrb1 to poly(A) + RNAs in splicing factor mutants. RNA co-immunoprecipitation experiments were performed with myc-tagged Gbp2, Hrb1 and Npl3 and GFP-tagged Tho2 and Thp2 in the indicated strains shifted to 37 °C for 30 min in three independent experiments. The co-precipitated poly(A) + RNA was detected by northern dot-blot hybridizations with a digoxigenin-labelled oligo d(T) 50 probe, set into relation with the total mRNA present in each strain and quantified relative to wild type. Error bars reflect s.d. ( b ) Functional Prp8 is required for proper association of Gbp2 and Hrb1 with Prp17. Co-IPs with myc-tagged Gbp2 or Hrb1 and Prp17-GFP were performed in wild type and prp8(908/988) cells; *, antibody chain. ( c ) Splicing is required for recruitment of Mex67 to Gbp2 and Hrb1. Western blots show the interaction between myc-tagged Gbp2, Hrb1 or Npl3 and Mex67-GFP in the indicated strains. All strains were shifted to 37 °C for 30 min. (*, antibody chain; L=lysate, W=final wash, E=eluate). Full size image Moreover, we find that the physical interaction of Gbp2 with the late splicing factor Prp17 is lost in prp8 ( 908/988 ) mutant cells and significantly reduced for Hrb1 ( Fig. 3b ). Prp8 contributes to conformational rearrangements necessary for the transition of the first to the second step of splicing and the significantly decreased association of the two SR proteins clearly emphasizes their splicing-dependent association with the spliceosome and spliced transcripts. Finally, if Gbp2 and Hrb1 are indeed absent from export competent mRNAs in splicing factor mutants, it would be expected that they would also not bind to the export receptor Mex67, since this protein should only be recruited to mature mRNAs upon the completion of splicing in order to signal their export competence. Indeed, co-IP experiments of Mex67 with either, Gbp2 or Hrb1 in the splicing factor mutants prp8 ( 908/988 ) and prp17 Δ show a loss of the interaction while the Mex67–Npl3 interaction is not significantly affected ( Fig. 3c ). These results indicate that Gbp2 and Hrb1 tightly associate with spliced transcripts on which they interact with the late spliceosome. Upon completion of splicing they provide a platform for the association of Mex67 molecules to the mature mRNAs. Gbp2 and Hrb1 interact with quality control factors An appealing model would be that Gbp2 and Hrb1 are recruited to the mRNA to bind additional molecules of Mex67 to support an efficient export of spliced transcripts. Thus, one would expect that the deletions of these two SR proteins would lead to specific export defects of spliced mRNAs. However, in situ hybridization experiments with an oligo d(T) 50 probe revealed no bulk mRNA export defects ( Fig. 4a ). Since the spliced transcripts are underrepresented in yeast (~5% of all genes contain introns) and a defect might not be visibly detectable, we further investigated specific mRNA localizations in in situ hybridization experiments with probes against specific intron-containing and intronless transcripts and found that neither of them are retained in gbp2 Δ or hrb1 Δ or the double knock out strain in contrast to the mex67-5 mutant ( Supplementary Fig. 4 ), indicating that Gbp2 and Hrb1 are not essential for mRNA export. 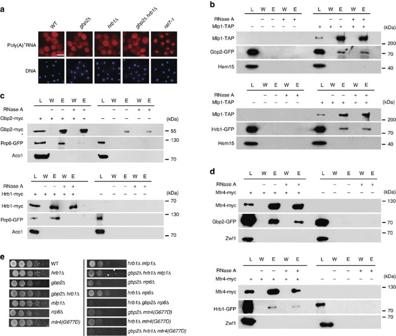Figure 4: Gbp2 and Hrb1 genetically and physically interact with quality control factors. (a) gbp2Δ and/or hrb1Δ do not have bulk mRNA export defects. The indicated strains are shown upon a 30 min temperature shift to 37 °C beforein situhybridizations with a Cy3-labelled oligo d(T)50probe were performed. The DNA is stained with 4′,6-diamidino-2-phenylindole (DAPI). Scale bar, 5 μm. (b) Physical interaction between Gbp2 or Hrb1 and the NPC component Mlp1. Co-IP experiments were performed with TAP-tagged Mlp1 and GFP-tagged Gbp2 or Hrb1. Log phase cells were lysed and split in two equal parts one of which was treated with RNase A (±). Hem15 served as a negative control. L,lysate; W, final wash; E, eluate. (c) Physical RNase sensitive interaction of Gbp2 and Hrb1 with the nuclear exosome component Rrp6. Co-IP experiments of Gbp2- and Hrb1-myc with Rrp6-GFP are shown from log phase cells. Aco1 served as negative control. (*, antibody chain). (d) Physical interactions between Gbp2 or Hrb1 and the TRAMP complex component Mtr4. Co-IP experiments were performed with myc-tagged Mtr4 and GFP-tagged Gbp2 or Hrb1. Zwf1 served as negative control. (e) gbp2Δ and/or hrb1Δ genetically interact with mlp1Δ, rrp6Δ and mtr4(G677D). Growth of mutants of the single genes and the gbp2Δ hrb1Δ double mutant (left) and in combination with mlp1Δ, rrp6Δ and a temperature-sensitive mutant of MTR4 (right) are shown. Cells were spotted in serial dilution onto FOA plates that select for the loss of a covering plasmid and incubated for 3 days at 25 °C. Figure 4: Gbp2 and Hrb1 genetically and physically interact with quality control factors. ( a ) gbp2Δ and/or hrb1Δ do not have bulk mRNA export defects. The indicated strains are shown upon a 30 min temperature shift to 37 °C before in situ hybridizations with a Cy3-labelled oligo d(T) 50 probe were performed. The DNA is stained with 4′,6-diamidino-2-phenylindole (DAPI). Scale bar, 5 μm. ( b ) Physical interaction between Gbp2 or Hrb1 and the NPC component Mlp1. Co-IP experiments were performed with TAP-tagged Mlp1 and GFP-tagged Gbp2 or Hrb1. Log phase cells were lysed and split in two equal parts one of which was treated with RNase A (±). Hem15 served as a negative control. L,lysate; W, final wash; E, eluate. ( c ) Physical RNase sensitive interaction of Gbp2 and Hrb1 with the nuclear exosome component Rrp6. Co-IP experiments of Gbp2- and Hrb1-myc with Rrp6-GFP are shown from log phase cells. Aco1 served as negative control. (*, antibody chain). ( d ) Physical interactions between Gbp2 or Hrb1 and the TRAMP complex component Mtr4. Co-IP experiments were performed with myc-tagged Mtr4 and GFP-tagged Gbp2 or Hrb1. Zwf1 served as negative control. ( e ) gbp2Δ and/or hrb1Δ genetically interact with mlp1Δ, rrp6Δ and mtr4(G677D). Growth of mutants of the single genes and the gbp2Δ hrb1Δ double mutant (left) and in combination with mlp1Δ, rrp6Δ and a temperature-sensitive mutant of MTR4 (right) are shown. Cells were spotted in serial dilution onto FOA plates that select for the loss of a covering plasmid and incubated for 3 days at 25 °C. Full size image Alternatively, Gbp2 and Hrb1 might have a function in nuclear quality control and the retention of pre-mRNAs. Thus, we investigated physical interactions between the two SR proteins and Mlp1 and found an RNase insensitive binding for both ( Fig. 4b ), uncovering a physical contact point of Gbp2 and Hrb1 with the NPC quality control factor Mlp1. Degradation of mRNAs that fail quality control involves the nuclear Rrp6-containing exosome [2] , [5] . We investigated a potential interaction between Rrp6 and Gbp2 or Hrb1 by co-IP studies and found a clear RNase sensitive physical interaction between Gbp2 or Hrb1 and Rrp6 ( Fig. 4c ). This indicates that Gbp2- and Hrb1-bound mRNAs are monitored by the nuclear exosome. The TRAMP complex has been suggested to mark RNAs for degradation, and we show that Gbp2 and Hrb1 physically interact with the TRAMP complex component Mtr4, which is not altered by the addition of RNase ( Fig. 4d ). These physical interactions are supported by genetic interactions between deletion mutants of GBP2 and/or HRB1 and mlp1 Δ, rrp6 Δ and a mutant of mtr4 ( Fig. 4e ). Gbp2 and Hrb1 control the nuclear retention of unspliced transcripts The physical and genetic interactions of Gbp2 and Hrb1 with the mRNA surveillance system strongly suggest a function in the nuclear quality control of spliced transcripts. To analyse this directly, we investigated whether the deletion of gbp2 Δ and hrb1 Δ, which does not lead to mRNA export defects ( Fig. 4a ), results in the opposite: The leakage of unspliced mRNAs into the cytoplasm. Therefore, we used a reporter leakage assay to detect the nuclear export of unspliced transcripts by measuring the expression of an intron-containing LacZ-reporter gene [29] . As shown in Fig. 5a we found that while the reporter-pre-mRNA was not translated at high levels in wild-type and npl3 Δ cells, leakage of unspliced mRNA into the cytoplasm was detected in mutants of the exosome component rrp6 Δ and the nuclear pore component mlp1 Δ, as shown earlier [29] . Strikingly, both gbp2 Δ and hrb1 Δ showed an even higher leakage rate of the unspliced transcript to the cytoplasm than the known quality control factors mlp1 Δ and rrp6 Δ ( Fig. 5a ), supporting a key role of these SR proteins in surveillance of spliced mRNAs. Since the deletion of GBP2 or HRB1 resulted also in very slight splicing defects ( Supplementary Fig. 2 ), we investigated whether splicing factor mutants in general would lead to a leakage of unspliced transcripts to the cytoplasm. However, this was not the case, neither a mutation in PRP43 , nor in PRP17 resulted in significant leakage ( Fig. 5a ). Furthermore, Gbp2 and Hrb1 associate with the THO- and TREX complex [20] . We investigated whether the deletion of MFT1 , which is part of both complexes and mutation of YRA1 , which is part of the TREX-complex would result in the enhanced transport of intron-containing transcripts to the cytoplasm, but we found no significant leakage ( Fig. 5a ), supporting a unique function of the SR proteins Gbp2 and Hrb1 in the surveillance of spliced transcripts. 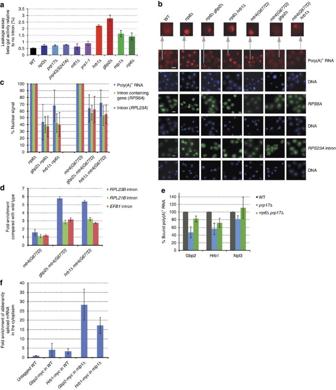Figure 5: Gbp2 and Hrb1 function in nuclear quality control of spliced transcripts. (a) Deletion ofGBP2andHRB1lead to an uncontrolled export of unspliced reporter mRNAs similar tomlp1Δ andrrp6Δ, but in contrast to the deletion of the other SR proteinNPL3or mutants of the splicing factorsPRP17andPRP43, the THO complex mutantmft1Δ and the mutated TREX componentYRA1. Strains were transformed with a leakage reporter plasmid to monitor the nuclear export of the encoded pre-mRNA. Shown is the β-galactosidase activity from an intron-containing compared with an intronlesslacZreporter gene. (b) Deletion ofGBP2orHRB1relieves the nuclear mRNA accumulation in an exosome and TRAMP complex mutant.In situhybridizations with a Cy3-labelled Oligo dT probe and DIG-labelled probes against the intron-containing transcriptRPS6Aand the intron ofRPS23Awere performed in the indicated strains, shifted to 37 °C for 3 h. The DNA was stained with DAPI. Scale bar, 5 μm. (c) Quantification of the nuclear signal shown in (b). 50 cells of each condition were quantified by using the Fiji software. (d) Increasing presence of intron-containing transcripts in the cytoplasmic fractions ofmtr4(G677D)cells and the double mutant strainsmtr4(G677D)gbp2Δ andmtr4(G677D)hrb1Δ. Cytoplasmic fractions were prepared and their RNA contents isolated. The intron sequences were amplified by qRT–PCR and the amount quantified. Their enrichment is depicted in comparison to the amount of introns detected in the cytoplasm of wild-type cells. (e) The reduced binding of Gbp2 and Hrb1 to poly(A)+RNA in splicing factor mutants seen inFig. 3ais relieved in the double mutantrrp6Δprp17Δ. Co-IP experiments were performed with myc-tagged Gbp2, Hrb1 and Npl3 in the indicated strains shifted to 37 °C for 30 min. The co-precipitated poly(A)+RNA was detected by northern dot-blot hybridizations with a digoxigenin-labelled oligo d(T)52probe and quantified relative to wild type. (f) Gbp2 and Hrb1 bind to aberrantly spliced mRNAs. RNA co-IP experiments with myc-tagged Gbp2 and Hrb1 from cytoplasmic fractions of wild type andmlp1Δ cells were performed. The co-precipitated poly(A)+RNA was analysed for the presence of the intron-containing lacZ leakage reporter. All experiments were performed three times independently. Error bars shown inaandc–ereflect s.d. Figure 5: Gbp2 and Hrb1 function in nuclear quality control of spliced transcripts. ( a ) Deletion of GBP2 and HRB1 lead to an uncontrolled export of unspliced reporter mRNAs similar to mlp1 Δ and rrp6 Δ, but in contrast to the deletion of the other SR protein NPL3 or mutants of the splicing factors PRP17 and PRP43 , the THO complex mutant mft1 Δ and the mutated TREX component YRA1 . Strains were transformed with a leakage reporter plasmid to monitor the nuclear export of the encoded pre-mRNA. Shown is the β-galactosidase activity from an intron-containing compared with an intronless lacZ reporter gene. ( b ) Deletion of GBP2 or HRB1 relieves the nuclear mRNA accumulation in an exosome and TRAMP complex mutant. In situ hybridizations with a Cy3-labelled Oligo dT probe and DIG-labelled probes against the intron-containing transcript RPS6A and the intron of RPS23A were performed in the indicated strains, shifted to 37 °C for 3 h. The DNA was stained with DAPI. Scale bar, 5 μm. ( c ) Quantification of the nuclear signal shown in ( b ). 50 cells of each condition were quantified by using the Fiji software. ( d ) Increasing presence of intron-containing transcripts in the cytoplasmic fractions of mtr4(G677D) cells and the double mutant strains mtr4 ( G677D ) gbp2 Δ and mtr4 ( G677D ) hrb1 Δ. Cytoplasmic fractions were prepared and their RNA contents isolated. The intron sequences were amplified by qRT–PCR and the amount quantified. Their enrichment is depicted in comparison to the amount of introns detected in the cytoplasm of wild-type cells. ( e ) The reduced binding of Gbp2 and Hrb1 to poly(A) + RNA in splicing factor mutants seen in Fig. 3a is relieved in the double mutant rrp6 Δ prp17 Δ. Co-IP experiments were performed with myc-tagged Gbp2, Hrb1 and Npl3 in the indicated strains shifted to 37 °C for 30 min. The co-precipitated poly(A) + RNA was detected by northern dot-blot hybridizations with a digoxigenin-labelled oligo d(T) 52 probe and quantified relative to wild type. ( f ) Gbp2 and Hrb1 bind to aberrantly spliced mRNAs. RNA co-IP experiments with myc-tagged Gbp2 and Hrb1 from cytoplasmic fractions of wild type and mlp1 Δ cells were performed. The co-precipitated poly(A) + RNA was analysed for the presence of the intron-containing lacZ leakage reporter. All experiments were performed three times independently. Error bars shown in a and c – e reflect s.d. Full size image To visualize this effect in vivo and to get additional and more direct evidence for the novel function of Gbp2 and Hrb1 in mRNA quality control by not using a single reporter mRNA, we performed in situ hybridization experiments. We analysed the nuclear accumulation of poly(A) + RNA, the intron-containing transcript RPS6A and the intron of RPL23A in mutants of the nuclear exosome, rrp6 Δ, and the TRAMP complex, mtr4 ( G677D ), in combination with gbp2 Δ or hrb1 Δ and found a ~50% reduced nuclear signal in the double mutants, with all three probes ( Fig. 5b,c ), which might be due to the fact that many spliced RNAs are highly expressed and increasingly accumulate in dependence of the time for which the mutant was shifted. This indicates that faulty RNAs that are prone to degradation accumulate in rrp6 Δ and mtr4 ( G677D ) and cannot escape from the nucleus in the presence of Gbp2 and Hrb1. However, in the absence of these SR proteins, such faulty mRNAs leak to the cytoplasm and the nuclear signal decreases. A third independent method was chosen to show leakage by separation of nuclear and cytoplasmic fractions of wild-type cells, mtr4 ( G677D ) and the double mutants mtr4 ( G677D ) gbp2 Δ and mtr4 ( G677D ) hrb1 Δ. First, the preparation of intact nuclei was verified by western blot analyses of Nop1 ( Supplementary Fig. 5a ). Second, the leakage of three different intron-containing transcripts into the cytoplasm was analysed by qRT–PCR analyses. As shown in Fig. 5d , intron sequences are slightly detectable in the cytoplasm of mtr4 ( G677D ) in comparison to wild-type cells. Interestingly, the number significantly increases in both double mutants mtr4 ( G677D ) gbp2 Δ and mtr4 ( G677D ) hrb1 Δ ( Fig. 5d ), reflecting an increased leakage of intron-containing transcripts into the cytoplasm. These data uncover a key function of Gbp2 and Hrb1 in mRNA surveillance of spliced transcripts. In other words, these data suggest that Gbp2 and Hrb1 detect aberrantly spliced transcripts and mediate their elimination. To investigate this more directly, we analysed whether the SR proteins in the absence of RRP6 , in which false transcripts should accumulate, would now show an increased binding to poly(A) + RNA. While the binding was reduced to ~50% for both SR proteins in splicing factor mutants ( Fig. 3a ), the binding increased in the rrp6 Δ prp17 Δ double mutant to 70–80% ( Fig. 5e and Supplementary Fig. 5b,c ), reflecting their binding to false transcripts. Since Npl3 is part of the these mRNP complexes as well, because it binds to bulk transcripts, its binding to poly(A) + RNA increased too ( Fig. 5e and Supplementary Fig. 5b,c ). Finally, we investigated the direct binding of Gbp2 and Hrb1 to a false transcript. We chose the lacZ leakage reporter transcript as an example, because it contains week splice sites [30] and it leaks to the cytoplasm in the MLP1 knock out strain in which leakage occurs ( Fig. 5a ; ref. 29 ). We separated the nucleus from the cytoplasm of wild-type and mlp1 Δ, co-immunoprecipitated the poly(A) + RNA bound to myc-tagged Gbp2 and Hrb1 from the cytoplasm and amplified the intron-containing lacZ transcript. As expected, the false transcript was very well detectable bound to both, Gbp2 and Hrb1 ( Fig. 5f ). These results show that Gbp2 and Hrb1 associate with false transcripts and cooperate with Mlp1 to retain them in the nucleus. Gbp2 and Hrb1 provide a switch for degradation and export The requirement of Gbp2 and Hrb1 in nuclear mRNA surveillance forced the question of how the SR proteins might mediate quality control. An attractive model would be that Gbp2 and Hrb1 function as regulators that recognize whether splicing is not completed in time. In this case they might allow the TRAMP complex to mark these faulty pre-mRNAs for degradation. In case splicing is completed in time Gbp2 and Hrb1 might instead bind to Mex67 to mark all correct mRNAs for export. If this model would be correct, one would expect that (a) the TRAMP complex can contact the spliceosome, (b) this contact is impaired in the absence of Gbp2 and Hrb1 and (c) Mex67-bound mRNAs should not bind to the TRAMP complex. An association of TRAMP with the spliceosome has been shown recently in yeast and in human cells [12] , [31] (and Fig. 6a ). Strikingly, this interaction is diminished in cells that lack Gbp2 or Hrb1 and lost in the double deletion strain ( Fig. 6a ), indicating that the presence of these SR proteins is necessary for proper TRAMP complex recruitment or stabilization of its binding to intron-containing pre-mRNAs. Further, co-IP experiments with Mex67-GFP show clear interactions with myc-tagged Gbp2 and Hrb1 ( Fig. 6b ), but not with Mtr4, suggesting that Mex67-bound mRNAs have already passed quality control. A similar result was also obtained when Mtr4 was immunoprecipitated and the co-precipitation of Gbp2 and Hrb1 with Mex67 was analysed ( Fig. 6c ). While Gbp2-myc and Hrb1-myc are detectable in western blots, a Mex67 association cannot be detected ( Fig. 6c ). These findings suggest that Gbp2 and Hrb1 can either bind to Mtr4 or to Mex67 and in this way direct transcripts to degradation or export. If so, one would expect that if proper quality control is prevented for example, in mutant MTR4 , the interaction of Gbp2 and Hrb1 with both, Mex67 and Mlp1 should be disturbed. This is indeed the case as shown in co-IP experiments ( Fig. 6d ). 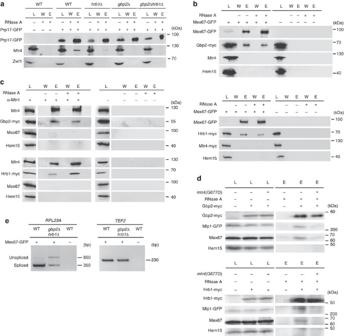Figure 6: Gbp2 and Hrb1 mediate quality control of spliced transcripts via TRAMP complex binding and upon surveillanceviaMex67 recruitment. (a) The TRAMP complex component Mtr4 interacts with the late splicing factor Prp17 and requires Gbp2 and Hrb1 for this interaction. Western blots of co-IP experiments of Mtr4 with Prp17-GFP are shown. Zwf1 served as a negative control. L, lysate; W, final wash; E, eluate (b) Gbp2 and Hrb1 in the Mex67-bound complex do not interact with Mtr4. Western blots of co-IP experiments of Gbp2-myc or Hrb1-myc with Mex67 and Mtr4 are shown. Hem15 served as a negative control. (c) In the Mtr4-bound complex Gbp2 or Hrb1 do not interact with Mex67. Western blots of co-IP experiments of myc-tagged Gbp2 and Hrb1 with Mtr4 and Mex67 are shown. Zwf1 served as a negative control. (d) The interaction of Gbp2 and Hrb1 with Mex67 and Mlp1 is disturbed inmtr4(G677D). Co-IP experiments with Mex67 and Mlp1-GFP were performed with myc-tagged Gbp2 and Hrb1 in wild-type andmtr4(G677D) cells upon a temperature shift to 37 °C for 30 min. (e) Mex67 binds to intron-containing mRNAs in the absence ofGBP2andHRB1. RNA co-IP experiments with Mex67-GFP were performed in wild-type andgbp2Δhrb1Δ. The co-precipitated poly(A)+RNA was isolated and used for RT–PCR experiments with an intron-containing (RPL23A) and an intronless (TEF2) transcript. Figure 6: Gbp2 and Hrb1 mediate quality control of spliced transcripts via TRAMP complex binding and upon surveillance via Mex67 recruitment. ( a ) The TRAMP complex component Mtr4 interacts with the late splicing factor Prp17 and requires Gbp2 and Hrb1 for this interaction. Western blots of co-IP experiments of Mtr4 with Prp17-GFP are shown. Zwf1 served as a negative control. L, lysate; W, final wash; E, eluate ( b ) Gbp2 and Hrb1 in the Mex67-bound complex do not interact with Mtr4. Western blots of co-IP experiments of Gbp2-myc or Hrb1-myc with Mex67 and Mtr4 are shown. Hem15 served as a negative control. ( c ) In the Mtr4-bound complex Gbp2 or Hrb1 do not interact with Mex67. Western blots of co-IP experiments of myc-tagged Gbp2 and Hrb1 with Mtr4 and Mex67 are shown. Zwf1 served as a negative control. ( d ) The interaction of Gbp2 and Hrb1 with Mex67 and Mlp1 is disturbed in mtr4 ( G677D ). Co-IP experiments with Mex67 and Mlp1-GFP were performed with myc-tagged Gbp2 and Hrb1 in wild-type and mtr4 ( G677D ) cells upon a temperature shift to 37 °C for 30 min. ( e ) Mex67 binds to intron-containing mRNAs in the absence of GBP2 and HRB1 . RNA co-IP experiments with Mex67-GFP were performed in wild-type and gbp2 Δ hrb1 Δ. The co-precipitated poly(A) + RNA was isolated and used for RT–PCR experiments with an intron-containing ( RPL23A ) and an intronless ( TEF2 ) transcript. Full size image Our model ( Fig. 7 ) would further suggest that intron-containing transcripts should be increasingly detectable bound to Mex67 in the gbp2 Δ hrb1 Δ strain as compared with the wild type. Therefore, we performed RNA co-IP experiments with Mex67-GFP in wild type and gbp2 Δ hrb1 Δ double knock out strains ( Fig. 6e and Supplementary Fig. 6 ). The purified poly(A) + RNA was subsequently used in RT–PCR experiments with an intron spanning primer set. Indeed, while Mex67 preferentially bound to the spliced RPL23A in wild type, it is clearly detectable on intron-containing RPL23A in the double-mutant gbp2 Δ hrb1 Δ ( Fig. 6e ). Taken together, our results support the conclusion that Gbp2 and Hrb1 function as surveillance factors for proper splicing and that they might act as switches between degradation and export. 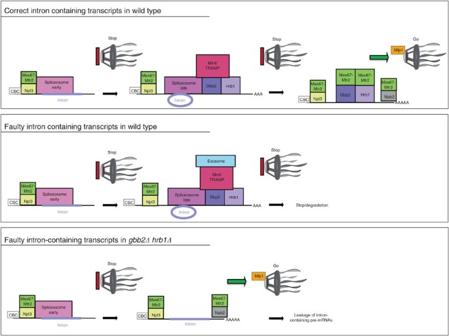Figure 7: Model for the nuclear quality control of spliced transcripts. Npl3 is recruited to the pre-mRNA early via RNA polymerase II (not shown), where it interacts with the mRNA cap-binding complex (CBC) and the early spliceosome. Npl3 associates with the heterodimer Mex67-Mtr2 to support export, but association of the spliceosome retains the mRNP. Gbp2 and Hrb1 bind at late steps of splicing to the spliceosome and recruit the TRAMP complex to the pre-mRNA. Faulty and unsplicible mRNAs are marked for degradation at the nuclear exosome (middle). On correct mRNPs, Gbp2 and Hrb1 recruit Mex67 to signal the export competence (top). In the absence of Gbp2 and Hrb1 (bottom) faulty pre-mRNAs exit the nucleus, because the surveillance system that monitors the completion of splicing is missing. Nab2 is involved in the 3′-end processing and recruits Mex67 upon completion. Proper coverage of the Npl3-, Gbp2, Hrb1- and Nab2-bound mature mRNA with Mex67 is monitored by Mlp1 at the NPC. Figure 7: Model for the nuclear quality control of spliced transcripts. Npl3 is recruited to the pre-mRNA early via RNA polymerase II (not shown), where it interacts with the mRNA cap-binding complex (CBC) and the early spliceosome. Npl3 associates with the heterodimer Mex67-Mtr2 to support export, but association of the spliceosome retains the mRNP. Gbp2 and Hrb1 bind at late steps of splicing to the spliceosome and recruit the TRAMP complex to the pre-mRNA. Faulty and unsplicible mRNAs are marked for degradation at the nuclear exosome (middle). On correct mRNPs, Gbp2 and Hrb1 recruit Mex67 to signal the export competence (top). In the absence of Gbp2 and Hrb1 (bottom) faulty pre-mRNAs exit the nucleus, because the surveillance system that monitors the completion of splicing is missing. Nab2 is involved in the 3′-end processing and recruits Mex67 upon completion. Proper coverage of the Npl3-, Gbp2, Hrb1- and Nab2-bound mature mRNA with Mex67 is monitored by Mlp1 at the NPC. Full size image To date a couple of factors important for nuclear mRNA surveillance have been identified that ensure the export of error-free mRNAs to the cytoplasm, where translation finally occurs. However, the underlying mechanisms and the coordination of mRNA quality control remained rather nebulous. In this work we have identified two shuttling SR proteins, Gbp2 and Hrb1, as novel key factors for the surveillance of spliced pre-mRNAs in yeast. Moreover, our results provide evidence for a model ( Fig. 7 ) in which these molecules resemble a checkpoint and function as switches to either stop faulty transcripts from being exported and initiate degradation, or to label correct mRNAs by recruitment of Mex67 for nuclear export. Yeast has been proven to be an excellent model organism for fundamental eukaryotic processes. The basic components of the splicing machinery are conserved between S. cerevisiae and mammalian cells [15] . However, in yeast only few transcripts are spliced and alternative splicing, which requires nuclear SR proteins and is prominent in higher eukaryotes has not been described in yeast. Besides their function in splicing, the shuttling SR proteins are thought to function as adapters for Mex67/TAP to promote export of mature mRNPs [32] . Yeast cells contain only the shuttling type of SR proteins (Npl3, Gbp2 and Hrb1) [17] , [18] , [19] . All three of them interact with Mex67 ( Fig. 1a , Supplementary Fig. 1a and ref. 16 ) and those mature mRNPs are exported into the cytoplasm. Npl3 associates with bulk mRNAs and is recruited early by RNA polymerase II [21] , [26] and might signal by recruitment of Mex67 that early processing events such as 5′-capping were properly executed. In fact, genetic and physical interactions have been described with the cap binding complex (CBC) components Cbp20 and Cbp80 (ref. 33 ). On spliced transcripts Npl3 participates in the recruitment of the early spliceosome [22] . At which time point Npl3 recruits Mex67 to these transcripts to support export is unclear and might involve protein modifications [5] , but even if Mex67 is already attached to Npl3 early, the association of the spliceosome most likely overbalances the export competence and might lead to the nuclear retention of the mRNP. Previous work has shown that the shuttling SR proteins Gbp2 and Hrb1 are recruited later during transcription via the THO complex [17] , [20] , through which they might initially contact bulk pre-mRNAs; however, we show here that their contact is stabilized and thus enriched on spliced transcripts by their physical interaction with late splicing factors ( Fig. 3b ). In fact, Gbp2 and Hrb1 have been purified earlier with the activated B complex (B act ) of the yeast spliceosome [28] and we detect binding of Gbp2 and Hrb1 to intron sequences ( Fig. 1d ) and splicing factors ( Figs 2b and 3b ), indicating that they are part of actively spliced mRNPs. This is further supported by the work of Tuck and Tollervey [27] , who identified a preferential association of Gbp2 on unspliced transcripts close to the 5′ region where intron sequences in yeast are mostly located by using the CRAC technique. Interestingly, a similar result was also shown for Mtr4 and Trf4, which might indicate an increased association of the TRAMP complex with unspliced pre-mRNAs, not least because of its potential involvement of degrading the intron sequences and its influence on splicing [11] , [12] , [27] . Furthermore, we show that tightened binding of Gbp2 and Hrb1 to spliced transcripts, mediated by the splicing complex is required for their subsequent Mex67 association ( Fig. 3c ) and their nucleo-cytoplasmic shuttling in association with spliced mRNAs ( Fig. 1b ). Additionally, we detect a significantly reduced binding of Gbp2 and Hrb1, but not of Npl3 or the THO complex components Tho2 and Thp2 to poly(A) + RNA in splicing factor mutants ( Fig. 3a ), revealing differences of Gbp2 and Hrb1 to the other SR protein Npl3 and the THO complex. As the THO complex is involved in the recruitment of Gbp2 and Hrb1 to bulk mRNAs, a possible explanation for the significantly reduced poly(A) + RNA association of Gbp2 and Hrb1 might be that their initial binding to bulk RNA is unstable and only their interaction with functional splicing factors ( Figs 2b and 3b ) stabilizes their binding on the transcript. Furthermore, inefficiently, or aberrantly spliced pre-mRNAs might have been rapidly degraded by the Gbp2–Hrb1-monitored TRAMP/exosome-degradation system, which might contribute to the reduced detection of poly(A) + RNAs associated with Gbp2 and Hrb1. Moreover, splicing defects further lead to a slowed 3′-end processing, which additionally triggers TRAMP-mediated degradation [5] . That these SR proteins are not simply adapters for Mex67 seems likely, because their deletions (even their double deletion) do not lead to mRNA export defects ( Fig. 4a ), but the opposite: the significant leakage of unspliced pre-mRNAs to the cytoplasm ( Figs. 5a–d and f ). This clearly shows that Gbp2 and Hrb1 are rather nuclear surveillance factors that retain unspliced transcripts in the nucleus. Moreover, we show that this function is unique to these SR proteins, because deletion or mutation of the THO- and TREX complex components MFT1 and YRA1 does not result in significant leakage of intron-containing transcripts into the cytoplasm ( Fig. 5a ). Furthermore, inhibition of splicing as shown in prp8(908/988) or prp17 Δ ( Supplementary Fig. 2 ) does not lead to leakage ( Fig. 5a ), supporting the outstanding function of Gbp2 and Hrb1 in the quality control of spliced transcripts. Once a faulty mRNA has been identified, Gbp2 and Hrb1 ensure that it is degraded in the nucleus by the TRAMP/exosome-degradation system ( Fig. 6a ). It is possible that, as suggested earlier, the extended association of TRAMP might thereby serve as a trigger for degradation [5] , but also models that involve phosphorylation or methylation of the SR proteins are possible. Our data further support a model in which upon correct splicing, mRNAs lose their association with TRAMP and are then not prone to degradation anymore. Instead Gbp2 and Hrb1 associate with Mex67, which seems to exclude their TRAMP-binding ( Fig. 6b,c ). Those mRNPs are now flagged with Mex67 that might signal the proper execution of splicing and indicate their export competence. Indeed, a transcriptome-wide atlas of RNP composition revealed that Gbp2 preferentially binds to 5′-regions of transcripts, similar to Mtr4 and Trf4, possibly because most of the intron sequences in yeast are close to the 5′-region, while the area of Mex67-binding is not restricted but rather distributed all over bulk transcripts, which include intronless mRNAs [27] . In our model we suggest that passing multiple quality control steps leads to the repeated association of Mex67 at different positions on the mRNA upon individual quality control checks ( Fig. 7 ). This model further suggests that Mex67 bound to Gbp2 and Hrb1 contacts Mlp1 at the NPC prior to export ( Fig. 7 ). This is supported by the fact that if quality control is not properly executed in defective MTR4 strains, the contact of Gbp2 and Hrb1 to Mex67 and Mlp1 is significantly reduced ( Fig. 6d ) and intron-containing transcripts, which might be exported via Npl3- and Nab2-bound Mex67 ( Fig. 7 ) are increasingly detected bound to Mex67 in the absence of GBP2 and HRB1 ( Fig. 6e ). Nab2 is a 3′-end processing factor, acting on bulk mRNAs, that has also been described as a Mex67 adapter protein, involved in mRNA surveillance via interaction with the NPC quality control factor Mlp1 (ref. 34 , 35 ). It seems likely that every maturation step is controlled, in this case the 3′-end processing step, and that the passage of each maturation ‘checkpoint’ might be labelled with the addition of one or more Mex67 molecules. The presence of Npl3- and Nab2-bound Mex67 might indeed be the reason for the observed leakage of unspliced transcripts in the absence of Gbp2 and Hrb1 ( Fig. 5a–d and f ). While in their presence faulty mRNAs are retained until they are degraded, those mRNAs cannot be channelled into the TRAMP/exosome-mediated degradation in the absence of Gbp2 and Hrb1. However, since they contain Npl3- and Nab2-bound Mex67 they might be exported like intron-free transcripts. In addition to Nab2, Npl3 has also been described to interact with Mlp1 (ref. 35 ). Here we show genetic and physical interactions of Gbp2 and Hrb1 with Mlp1 ( Fig. 4 ). It is possible that all these interactions are not direct but rather mediated via Mex67. Therefore, it is interesting to envision that Mlp1 might functions as a ticket controller that checks for the coverage of these mRNA-binding proteins with Mex67 and on spliced transcripts simply more tickets might be necessary to pass this final quality control checkpoint. Plasmids and yeast strains All yeast strains used in this study are listed in Supplementary Table 1 , plasmids in Supplementary Table 2 and oligonucleotides in Supplementary Table 3 . Strains were cultivated in standard media at 25 °C. All growth tests are shown in 10-fold serial dilution starting with ~10 5 cells per drop. Construction of plasmids and yeast strains: chromosomal deletion mutants and the generation of chromosomal tags were generated by transformation of PCR-amplified DNA fragments for homologous recombination. The haploid knock-out strains were verified by PCR. For C-terminal tagging the myc-insertion cassette was amplified by PCR from the plasmid pHK492 for homologues recombination. All created double- and triple-mutant strains were generated by crossing of the respective parental strains of the opposite mating type in the presence of a rescue plasmid, encoding for one of the deleted or mutated genes bearing an URA3 marker. Diploid strains were then sporulated and subjected to tetrad dissection. All spores were analysed by genetic markers and gene deletions were verified via PCR. HKY428, HKY433, HKY631 and HKY1144 were identified in the EMS mutagenesis screen as temperature-sensitive mutants. The respective point mutations were analysed by PCR amplification of the respective gene and identified by sequencing of the genomic DNA. Construction of myc-NPL3 : the 9x-myc tag sequence was amplified from the plasmid pHK493. Correct integration of the myc-tag was verified by PCR amplification of the genomic DNA and the protein expression was controlled by western blot using anti-myc-antibodies. Gbp2 c -GFP (pHK571) was sub-cloned within a Not I/ Kpn I fragment from pHK431 into a 2μ URA3 vector. The PRP17–GFP plasmid was created by cloning the PRP17 PCR fragment with restriction sites Xho I and Bam HI into a GFP vector with an ADH promoter, resulting in pHK892. All other plasmids created in this study were sub-cloned into a different vector system to obtain specific selectable marker, such as a GFP-tag fusion or to express the gene from the strong ADH promoter or an inducible GAL1 promoter. All other strains and plasmids can be found in the Supplementary Tables 1 and 2 . Co-immunoprecipitation experiments Log phase yeast cells were lysed at a density of OD 600 ~1 in PBSKMT buffer (1 × PBS, 3 mM KCl, 2.5 mM MgCl 2 , 0.5% Triton X-100, including protease inhibitors from Roche and Sigma). The supernatant was split into two equal parts (±addition of 200 μg ml −1 RNase) and incubated for 3–4 h at 4 °C with IgG sepharose beads, Protein G sepharose or G Plus agarose beads, conjugated to the respective antibodies (2 μg). After washing with PBSKMT buffer, samples were analysed on western blots with the indicated antibodies (GFP (Santa Cruz) 1:500; myc (Santa Cruz) 1:750; Zwf1 (Sigma) 1:50,000; Hem15 (R. Lill) 1:5,000; Aco1 (R. Lill) 1: 2,000; Mtr4 (P. Linder) 1:2,000; Mex67 (C. Dargemont) 1:50,000). 30 μl of each 800 μl lysate and final 30 μl wash sample were loaded. Upon the IPs, the beads were mixed with 30 μl SDS sample buffer and subsequently loaded onto an SDS gel for the western blot analyses. All western blots shown in one figure are from one gel and the lanes were excised in order to show multiple proteins. The sizes of molecular weight marker bands are indicated. The complete scans of the most important western blot analyses are shown in Supplementary Fig. 7 . EMS mutagenesis and screening Ethyl methane sulphonate (EMS)-mutagenized wild-type cells (HKY36) were screened for temperature sensitivity at 37 °C and nuclear mislocalization of Gbp2 c -GFP (pHK571). The mutated genes of the temperature sensitive mutants were identified by complementation with plasmid libraries [36] . GFP localization Green fluorescent protein (GFP)-tagged proteins were analysed in the fluorescence microscope upon a 1-min fixation in 2.5% formaldehyde and subsequent washing once with 0.1 M phosphate buffer pH 6.5 and once with P-solution (0.1 M phosphate buffer pH 6.5 and 1.2 M sorbitol). RNA co-immunoprecipitation experiments Yeast cells were grown at 25 °C in selective medium to a density of 4 × 10 7 cells per ml. The cells were collected, washed with 1 × TBS and resuspended in RNA-IP buffer (25 mM Tris–HCl, (pH 7.5), 100 mM KCl, 0,2% ( v / v ) Triton X-100, 0.2 mM PMSF, 5 mM DTT, 10 units RiboLock RNase Inhibitor (Thermo Scientific)). One cell pellet volume of glass beads, 1.5 volumes of RNA-IP buffer including protease inhibitor cocktails (Sigma-Aldrich and Roche Applied Science) were added. Cells were lysed by vigorous vortexing for 25 s and 4 m s −1 using the FastPrep-24 instrument (MP Biomedicals). For DNaseI digestion 800 μl lysate was incubated with 15 μl (40 Kunitz units) DNaseI (Qiagen) at 30 °C for 30 min. The co-immunoprecipitation experiments were performed at 4 °C for 3 h by incubating lysates with 20 μl of Protein G sepharose beads (Amersham Biosciences) conjugated to monoclonal c-myc (9E10)-antibody (Santa Cruz) or GFP-Trap-beads (ChromoTek). The beads were washed five times with RNA-IP buffer and the RNA was eluted in 100 μl DEPC-treated ddH 2 O during incubation at 65 °C for 10 min. The RNA eluate was purified via phenol–chloroform extraction followed by an ethanol precipitation. The RNA was finally eluted in 10 μl of DEPC-treated ddH 2 O. 100 μl of the lysate was processed in parallel to obtain a total input sample for microarray, northern dot blots and qRT–PCR analyses. Microarray analyses The RNA probes from RNA co-immunoprecipitations were qualitatively analysed by Experion (Biorad). One microgram of RNA was amplified using the Message Amp II mRNA Amplification kit (Ambion). Four micrograms of an RNA sample were reverse transcribed into Cy3- or Cy5-labelled cDNA using the Amersham CyScribe cDNA Post-labelling kit (GE Healthcare). Unincorporated nucleotides were removed following the manufacturers protocol of illustra CyScribe GFX Purification kit (GE Healthcare). Yeast microarray slides (Y6.4k6; University Health Network Microarray Centre, Toronto, Canada) were pre-hybridized at 55 °C for 30 min in 5 × SSC, 0.1% SDS and 1% bovine serum albumin and rinsed five times with water. The slides were dried by spinning at 1,500 r.p.m. for 3 min. Labelled probes were supplemented with 3 μl of yeast tRNA (10 mg ml −1 ) and 3 μl of denatured salmon sperm DNA (10 mg ml −1 ). Probes were concentrated in a speed vac to a final volume of 26 μl and supplemented with 4 μl 2% bovine serum albumin and 10 μl 20 × SSC before they were spotted onto a microarray slide. The hybridization was carried out for 16 h at 55 °C in a hybridization chamber. After removal of the HybriSlipTM Hybridization Cover (Sigma-Aldrich) the slides were washed with agitation three times in 1x SSC buffer containing 0.1% SDS, two times with 1 × SSC buffer and once in ddH2O. Arrays were dried by centrifugation in 50 ml Falcon tubes for 3 min at 1,500 r.p.m. Fluorescence intensities were monitored by using the scanner ScanArray Express (PerkinElmer Life Sciences) system and the Agilent Microarray scanner. The microarrays, which contain two spots for each gene, were inspected for labelling and hybridization quality. Individual microarrays were made comparable by normalizing their expression levels using the quantile method [37] , separately for the data related to Gbp2, Hrb1 or Npl3. Normalized expression levels were log2-transformed for variance stabilization and the spot-doublet of each gene was averaged. In order to merge the data of the two replicates, a joint gene-wise fold change between lysate and eluate was derived using the linear models proposed by Smyth [38] . The regression coefficients of the linear model can be regarded as the log2-fold changes (FC) between two groups of samples. Genes that were enriched in the eluate by a factor of 1 were regarded for further enrichment analyses. With this criterion, 287 genes were selected for Gbp2, 657 for Hrb1 and 455 for Npl3. Among the genes selected for Gbp2, 34/287 (12%) were introns, compared with 186/6,008 (3%) of introns among the non-selected genes. In terms of the odds ratio (OR), a 4.2-fold enrichment was thus observed for Gbp2 (95% CI: (2.8, 6.2)), which is significant according to Fisher’s exact test ( P <0.01). A significant enrichment of introns was also detected for Hrb1 ( P <0.01). In detail, 38/657 (6%) of selected genes were introns, in contrast to 182/5,638 (3%) of introns in the non-selected genes. This transfers to an OR of 1.8 (95% CI: (1.2, 2.7)). No enrichment was observed for Npl3 ( P =0.14). For this protein, only 10 (2%) of 455 selected genes were introns, compared with 210 (4%) introns among 5,840 non-selected genes, which transfers to an OR of 0.6 (95% CI: (0.3, 1.1)). The above enrichments and non-enrichment, respectively, were also observed in the individual replicates of the related proteins. ORs for joint and individual analyses are depicted in Fig. 1c . All analyses were performed using the software R (version 2.15, www.r-project.org ). Normalization and the linear model were conducted using the R-package ‘limma’. Reverse transcription and quantitative PCR (qRT-PCR) One microgram of RNA from the RNA co-immunoprecipitation experiments was reversed transcribed using oligo(dT) primers and the Omniscript kit (Qiagen, Hilden, Germany) or Maxima Reverse Transcriptase (Thermo Scientific). For the untagged wild-type controls the whole eluate was used. qPCR was performed in a Mx3000P Real-Time PCR system (Stratagene) or with the Rotor-Gene (Qiagen) for 40 cycles at an annealing temperature of 57–60 °C. With the GoTaq master mix (Promega) and a primer concentration of 0.2 μM the PCR reaction were started following the manufacturers instruction. The qRT–PCR analyses were done for three independent experiments and each gene amplification was performed in triplicates. In situ RNA hybridization Localization of poly(A) + RNA by in situ hybridization were performed by using a Cy3-labelled oligo d(T) probe. Specific RNA probes were generated with incorporated digoxigenin (DIG). For synthesis of DIG-UTP -abelled RNA probes, 250 ng purified PCR templates were generated including a T7 transcription site on an antisense strand. In vitro transcription of the antisense RNA was performed using T7 RNA polymerase (Fermentas) and DIG-UTP RNA labelling Mix (Roche) according to the standard protocol. DIG-labelled antisense transcripts were precipitated with 1/4th 4 M LiCl, 1 μl glycogen and 2.5 vol. EtOH and resuspended in 0.5 × TE/formamide/hybmix (50% formamide, 5 × SSC, 5 × Denhardts, 250 μg ml −1 tRNA, 500 μg ml −1 salmon sperm DNA, 50 μg ml −1 heparin, 2.5 mM EDTA (pH 8.0), 0,1% ( v / v ) Tween 20). For RNA in situ hybridization cells were grown to 2 × 10 7 cell per ml at 25 °C and shifted to 37 °C for the indicated time. Cells were fixed by adding formaldehyde to a final concentration of 4% and incubated for 30 min at 37 °C. Cells were collected and washed twice with 0.1 M phosphate buffer (pH 6.5) and once with P-solution. Cells were zymolase-treated, permeabilized and then pre-hybridized with hybmix (4 × SSC; 5 mM EDTA (pH 8.0); 0,1% Tween 20; 1 × Denhardt's solution (1% Ficoll, 1% polyvinylpyrrolidone, 1% bovine serum albumin); 0.1% heparin) for 1 h on a polylysine-coated slide. After hybridization over night at 37 °C with the respective digoxigenin-labelled RNA probe, cells were washed with 0.5–2 × SSC. Cells were blocked in antibody-blocking buffer for 1 h. A sheep anti-digoxigenin Fab-FITC antibody (Roche) was used at a 1:200 dilution and incubated over night at 4 °C. After washing with Aby wash I buffer (0.1 M Tris–HCl (pH 9.0), 0.15 M NaCl) nuclei were stained with DAPI. Microscopy studies were performed with a Leica AF6000 microscope and pictures were obtained by using the Hamamatsu 1394 ORCA-ERA camera and the LAS AF 1.6.2 software (Leica). Northern blot experiments For the radioactive northern blot experiments equal amounts of total RNA were transferred onto a Hybond N+ nylon membrane (GE Healthcare) and UV crosslinked (254 nm, 120,000 μJ cm −2 ). Afterwards, the membrane was pre-hybridized for 4 h in pre-hybridization buffer (0.5 M sodium phosphate buffer (pH 7.5), 7% ( w / v ) SDS, 1 mM EDTA, 50 μg ml −1 salmon sperm DNA) and hybridized overnight in pre-hybridization buffer plus 32 P-labelled GFP or ADH1 probe at 55 °C. The membrane was washed three times in 0.04 M sodium phosphate (pH 7.2) and 0.1% ( w / v ) SDS for 10 min each. The signal intensity was quantified using a PhosphorImager (FLA-3000, Fujifilm). For the northern dot blot experiments, equal amounts of total RNA and protein-bound RNAs from the eluate were spotted onto a Hybond N + nylon membrane (GE Healthcare) and UV crosslinked (254 nm, 120,000 μJ cm −2 ). Upon pre-hybridization for 1 h, the membrane was incubated with a DIG-labelled oligo d(T) 52 probe and incubated over night at 45 °C for hybridization. The membrane was washed one time in 2 × SSC, 0,1% ( w / v ) SDS and one time in 1 × SSC, 0,1% ( w / v ) SDS for 15 min at room temperature. Final washing steps were performed twice in 0.5 SSC, 0.1% ( w / v ) SDS for 15 min at 45 °C. After washing the DIG labelling was detected using the DIG High Prime DNA labelling and Detection starter kit II kit (Roche) according to the manufacturer’s instructions. Signal intensities of dot blots were monitored and quantified using the chemiluminescence imaging system Fusion FX7 and Fusion-Capt software (Peqlab). All northern blot analyses were done at least three times. Leakage assay Experiments were essentially performed as described [29] : Cells were grown at 25 °C to a density of OD 600 0.5-0.8 in the appropriate medium. Cells were induced with galactose for 1.5 h and shifted to 37 °C for 30 min in galactose containing media. Cells were washed in Z-buffer (100 mM phosphate buffer (pH 7.0), 10 mM KCl, 1 mM MgSO 4 ) and resuspended in 300 μl Z-buffer. The cells were lysed using the freeze–thaw method. Afterwards 700 μl Z-buffer supplemented with 2,7 mM ß-Mercaptoethanol and 160 μl of o -nitrophenyl-β- D -galactopyranoside solution (4 mg ml −1 ) was added to the lysate and the mixture was incubated at 30 °C for the respective time. The reaction was stopped with 400 μl 1 M Na 2 CO 3 . β-galactosidase activity was assayed by measuring hydrolysis of the chromogenic substrate at OD 420 . The leakage assay was done for each strain three times. Nucleo-cytoplasmic fractionation Log phase yeast cultures (50 ml) were collected and washed with 2 mM DTT. Pellets were resuspended in 5 ml 1 M sorbitol and 1 mM DDT containing YPD medium including 25 mg of zymolase and incubated at 30 °C for 20 min. Spheroplasts were collected by centrifugation at 2,500 r.p.m. for 3 min, washed once in 1 M sorbitol containing YPD medium and further incubated for 20 min before the spheroplasts were finally pelleted and resuspended in ice-cold phosphate buffer (PVP-buffer: 8% ( w / v ) polyvinylpyrrolidone, 1 mM MgCl 2 , 20 mM K-phosphate buffer (pH 6.5)) containing 0,03% ( w / v ) Triton X-100. Cells were mixed with PVP buffer including 0.6 M saccharose and opened by douncing. The lysates were pipetted onto PVP buffer with 0.45 M saccharose and centrifuged at 4,500 r.p.m. in a swing-out rotor. The top fraction (~300 μl) contained the cytoplasmic fraction. The nuclei were in the bottom fraction. Accession codes: Microarray data have been deposited in the Gene Expression Omnibus (GEO) data base with the accession no. GSE52808 . How to cite this article: Hackmann, A. et al. Quality control of spliced mRNAs requires the shuttling SR proteins Gbp2 and Hrb1. Nat. Commun. 5:3123 doi: 10.1038/ncomms4123 (2014).